Photo-generated dinuclear {Eu(II)}2active sites for selective CO2reduction in a photosensitizing metal-organic framework Photocatalytic reduction of CO 2 is a promising approach to achieve solar-to-chemical energy conversion. However, traditional catalysts usually suffer from low efficiency, poor stability, and selectivity. Here we demonstrate that a large porous and stable metal-organic framework featuring dinuclear Eu(III) 2 clusters as connecting nodes and Ru(phen) 3 -derived ligands as linkers is constructed to catalyze visible-light-driven CO 2 reduction. Photo-excitation of the metalloligands initiates electron injection into the nodes to generate dinuclear {Eu(II)} 2 active sites, which can selectively reduce CO 2 to formate in a two-electron process with a remarkable rate of 321.9 μmol h −1 mmol MOF −1 . The electron transfer from Ru metalloligands to Eu(III) 2 catalytic centers are studied via transient absorption and theoretical calculations, shedding light on the photocatalytic mechanism. This work highlights opportunities in photo-generation of highly active lanthanide clusters stabilized in MOFs, which not only enables efficient photocatalysis but also facilitates mechanistic investigation of photo-driven charge separation processes. The ever-increasing atmospheric carbon dioxide (CO 2 ) level due to fossil fuel consumption raises growing concerns about global warming [1] , [2] . Therefore, developing new technology for CO 2 capture and conversion is receiving considerable research interest. In this context, photocatalytic reduction of CO 2 into renewable fuels is a promising strategy for solar-to-chemical energy conversion by using artificial photosynthetic systems [3] , [4] , [5] . This approach not only uses CO 2 as C 1 feedstock but also allows harvesting energy from sunlight, helping the transition towards a more sustainable energy source. During the last few decades, diverse inorganic semiconductors have been developed for carbon fixation, such as TiO 2 [6] , CdS [7] , ZnO [8] , and ZnGa 2 O 4 [9] , which were synthesized as photocatalysts to reduce CO 2 . However, the efficiencies of these materials are limited by their large band gaps, low densities of active sites on surfaces, and fast recombination rates of photo-generated electron–hole pairs [10] , [11] , [12] , [13] . Therefore, exploring new photocatalysts with enhanced efficiency for solar-driven CO 2 reduction is highly desirable. Metal-organic frameworks (MOFs), one type of crystalline porous hybrid materials, have attracted widespread attention due to their tailorable chemistry, uniform but tunable porosity, and high surface areas [14] , [15] , [16] , [17] , [18] . Up to now, great efforts have been dedicated to the synthesis and catalytic applications of porous MOFs. Recently, several MOFs have been taken as heterogeneous catalysts for photocatalytic reduction of CO 2 , including NH 2 -MIL-125(Ti) [19] , NH 2 -UiO-66(Zr) [20] , and porphyrin-MOFs [3] , [21] , some of which adopt the connecting metal clusters as the active sites. These metal clusters play a significant role on the photocatalytic activity of catalysts in photoreduction of CO 2 . Studies on lanthanide chemistry have shown that Eu(II) ion is highly active in reductive conversions [22] , [23] . We envisioned that introducing Eu(III) clusters as metal connecting nodes in MOFs followed up with photo-activation can generate isolated Eu(II) active cluster sites for CO 2 reduction. On the other hand, ruthenium-polypyridine compounds are often used as photosensitizer for photocatalytic CO 2 reduction due to their tremendous oxidation and reduction power and extended lifetimes of their excited states [24] , [25] , [26] . Studies by García et al. [27] and Majima et al. [28] revealed that the organic ligands in MOFs can serve as antenna for the metal clusters. Photoexcited electron transfer from ligands to catalytic centers is also observed. These previous studies lead us to hypothesize that integrating Ru-polypyridine photosensitizers into Eu cluster-based MOFs will be a promising strategy to enhance the catalytic activities on CO 2 reduction under visible-light irradiation. Here, we design an Eu-Ru(phen) 3 -MOF (phen = phenanthroline) by integrating the triangular Ru(phen) 3 -derived tricarboxylate ligand as photosensitizer into Eu-MOF with Eu 2 (μ 2 -H 2 O) secondary building units (SBUs). Interestingly, the Eu-Ru(phen) 3 -MOF exhibits visible-light-driven selective CO 2 photoreduction to formate with a remarkable rate of 321.9 μmol h −1 mmol MOF −1 . Noteworthily, such a self-assembled Eu-Ru(phen) 3 -MOF is the solitary example that exhibits a high efficiency for selective CO 2 photo-reduction in the family of Ln-MOFs. Time-resolved photoluminescence (PL) spectroscopy combined with femtosecond transient optical absorption spectroscopy confirms that charge transfers from Ru photocenters to Eu-O cluster on a time scale of 1 to 300 ns. Moreover, in situ electron paramagnetic resonance (EPR) study clearly indicates that after accepting of photoexcited electrons from metalloligand, the Eu(III) 2 clusters become active catalytic centers for the photoreduction of CO 2 . Synthesis and structural determination of Eu-Ru(phen) 3 -MOF The triangular Ru(phen) 3 -derived tricarboxylate acid metalloligand (H 3 L ) was prepared from 1,10-phenanthroline in a multistep sequence in a 73% overall yield, as shown in Fig. 1 (Supplementary Figs. 1 – 7 and Supplementary Methods). The resultant Eu-Ru(phen) 3 -MOF formulated as [Eu 2 (μ 2 -H 2 O)(H 2 O) 3 (L) 2 ]·(NO 3 ) 2 ·(2-FBA − ) 2 ·(H 2 O) 22 was synthesized by a reaction of Eu(NO 3 ) 3 ·6H 2 O, H 3 L , and 2-fluorobenzoate (2-FBA) in dimethylformamide (DMF) at 105 °C for 70 h (small light red block-shaped crystals in 44% yield). Single-crystal X-ray crystallographic study with synchrotron radiation reflected that the Eu-Ru(phen) 3 − MOF crystallize in a orthorhombic crystal system with space group of I 222 . The MOF adopts a structure of twofold interpenetrated coordination networks. Within each of the framework, the propeller-like metalloligands with D 3 symmetry and six-connected (6-c) [Eu 2 (μ 2 -H 2 O)(H 2 O) 3 (-COO − ) 6 ] SBUs (Fig. 2a ) linked to each other alternately to generate a three-dimensional (3D) framework containing one-dimensional 16 × 31 Å channels along the [010] direction (Fig. 2b, c ). The three-connected (3-c) metalloligand and the 6-c {Eu(III)} 2 cluster (Fig. 2d ) are linked together, leading to a (3,6)-connected scu -type topology with the (4•6 2 ) 2 (4 2 •6 9 •8 4 ) point symbol (Supplementary Fig. 8 ). Two sets of the symmetric net interpenetrated into each other, resulting in a twofold interpenetrated structure (Fig. 2e ). There are two types of interconnected channels in the Eu-Ru(phen) 3 -MOF structure: one is a continuous channel along the [011] direction, with window dimensions of 15 × 20 Å, and the other one with smaller aperture is along the [111] direction (Supplementary Fig. 9 ). As depicted in Fig. 2e, f , the π–π stacking interactions between metalloligands stabilized the adjacent interpenetrated frameworks. The void space in the MOF was calculated to be 74.5% by PLATON [29] . The amount of nitrogen gas adsorption of Eu-Ru(phen) 3 -MOF at 77 K is far less than that predicted from the structure (Supplementary Fig. 10 ) due to distortion of the framework during drying process (Supplementary Note 1 ) [30] , [31] . Based on thermogravimetric analysis (TGA) (Supplementary Fig. 11 ) and charge balance, there are two NO 3 − and two 2-FBA anions in the channel of the Eu-Ru(phen) 3 -MOF. Fig. 1 Synthesis of H 3 L . Chemical structure of the tricarboxylate metalloligand used in the synthesis of Eu-Ru(phen) 3 -MOF. (i) HNO 3 , H 2 SO 4 , KBr, NaOH, 90 °C, 96% yield; (ii) 4-carboxybenzaldehyde, HAc, 100 °C, NH 4 Ac, 120 °C, 88% yield; (iii) RuCl 3 ·3H 2 O, EG, 180 °C, KFP 6 (aq), NaOH(aq), THF, EtOH, 80 °C, 87% yield Full size image Fig. 2 X-ray crystal structure of Eu-Ru(phen) 3 -MOF. a Stick/polyhedra model structure of the metalloligand. b Stick model representation of a single 3D framework viewed along the [010] direction showing the 1D channels c with window dimensions of 31 × 16 Å. d Ball-and-stick model of [Eu 2 (μ 2 -H 2 O)(H 2 O) 3 (-COO − ) 6 ] building unit in Eu-Ru(phen) 3 -MOF. e Stick model showing the interpenetrated frameworks in Eu-Ru(phen) 3 -MOF and f the two neighboring networks stabilized by the π–π stacking interactions Full size image Photocatalytic CO 2 reduction The photocatalytic CO 2 reduction activity was tested under visible-light irradiation (420 nm < λ < 800 nm) by using Eu-Ru(phen) 3 -MOF as heterogeneous photocatalyst and triethanolamine (TEOA) as sacrificial agent (Supplementary Fig. 12 ). The concentration of formate HCOO − product in the liquid phase was quantified by using ion chromatograph. As shown in Fig. 3a , under continuous visible-light illumination, formate production exhibits a time-dependent increase. 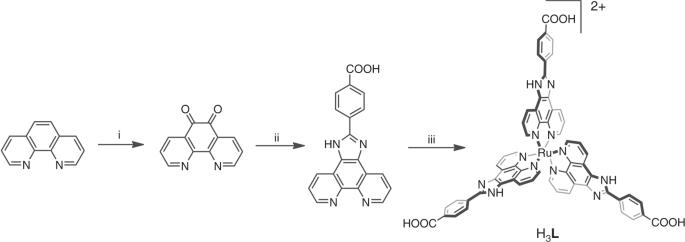Fig. 1 Synthesis of H3L. Chemical structure of the tricarboxylate metalloligand used in the synthesis of Eu-Ru(phen)3-MOF. (i) HNO3, H2SO4, KBr, NaOH, 90 °C, 96% yield; (ii) 4-carboxybenzaldehyde, HAc, 100 °C, NH4Ac, 120 °C, 88% yield; (iii) RuCl3·3H2O, EG, 180 °C, KFP6(aq), NaOH(aq), THF, EtOH, 80 °C, 87% yield 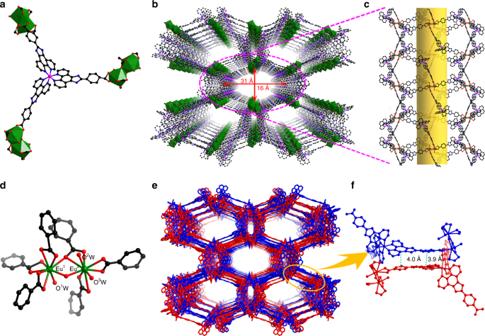Fig. 2 X-ray crystal structure of Eu-Ru(phen)3-MOF.aStick/polyhedra model structure of the metalloligand.bStick model representation of a single 3D framework viewed along the [010] direction showing the 1D channelscwith window dimensions of 31 × 16 Å.dBall-and-stick model of [Eu2(μ2-H2O)(H2O)3(-COO−)6] building unit in Eu-Ru(phen)3-MOF.eStick model showing the interpenetrated frameworks in Eu-Ru(phen)3-MOF andfthe two neighboring networks stabilized by the π–π stacking interactions 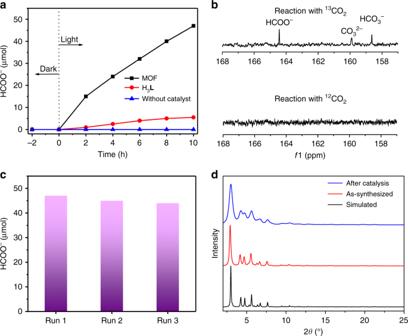Fig. 3 Photocatalytic CO2reduction performance.aTime profiles of HCOO−produced catalyzed by Eu-Ru(phen)3-MOF or H3Lor without catalyst under irradiation with a Xe lamp (420–800 nm).bThe13C NMR spectrum of products in liquid phase after reacting with13CO2and12CO2, respectively.cThe amount of HCOO−produced for reusing three times. Samples were recovered after each cycle and reused under identical reaction conditions.dPXRD patterns for as-synthesized Eu-Ru(phen)3-MOF and after photocatalytic reaction, showing its well-retained structure during the catalysis The amount of generated HCOO − reached 47 μmol in 10 h with the average formation rate of HCOO − of 321.9 μmol h −1 mmol MOF −1 (mmol MOF calculated from its SBUs, Supplementary Table 1 ). This value is higher than those of previous catalyst bast on MOF materials, such as NH 2 -MIL-125(Ti), NH 2 -UiO-66(Zr), and PCN-222 under similar conditions (the formation rates of HCOO − for these photocatalysts are 26.5, 46.3, and 143.5 μmol h −1 mmol MOF −1 , respectively) [19] , [20] , [21] , and some visible-light responsive semiconductors [32] , [33] . The higher photocatalytic activity should be attributed to the introduction of a photosensitizing and efficient light-harvesting Ru(phen) 3 moiety in this system. In addition, no CO or H 2 or CH 4 products in the gas or liquid phases was observed (Supplementary Figs. 13 and 14 ), suggesting that Eu-Ru(phen) 3 -MOF has high selectivity in reducing CO 2 to formate. The control experiments showed that no HCOO − was produced either without Eu-Ru(phen) 3 -MOF, TEOA, or in dark (Supplementary Fig. 15a ). To evaluate the photocatalytic stability, recycling experiments of photocatalytic CO 2 reduction in MeCN/TEOA ( v:v = 20:1) were performed (Supplementary Fig. 15b ). As shown in Fig. 3a , after 10 h illumination, the HCOO − amount was about 47 μmol and no noticeable degradation after three consecutive reactions (Fig. 3c ). Meanwhile, the PXRD patterns after photocatalytic reactions match well with those of as-prepared sample, suggesting the stability of Eu-Ru(phen) 3 -MOF after photocatalytic reaction (Fig. 3d ). The scanning electron microscope (SEM) images show that morphology of the Eu-Ru(phen) 3 -MOF changed after photocatalytic reaction as a result of mechanical stirring (Supplementary Fig. 16 ). Moreover, inductively coupled plasma-mass spectrometry (ICP-MS) results indicates <0.1% metal leaching to the solution after photocatalytic reaction of 10 h, confirming the stability of Eu-Ru(phen) 3 -MOF in photocatalysis. Fig. 3 Photocatalytic CO 2 reduction performance. a Time profiles of HCOO − produced catalyzed by Eu-Ru(phen) 3 -MOF or H 3 L or without catalyst under irradiation with a Xe lamp (420–800 nm). b The 13 C NMR spectrum of products in liquid phase after reacting with 13 CO 2 and 12 CO 2 , respectively. c The amount of HCOO − produced for reusing three times. Samples were recovered after each cycle and reused under identical reaction conditions. d PXRD patterns for as-synthesized Eu-Ru(phen) 3 -MOF and after photocatalytic reaction, showing its well-retained structure during the catalysis Full size image The control experiment using 13 CO 2 as reactant was studied to validate the source of HCOO − product, and the generated H 13 COO − was detected by 13 C NMR spectroscopy. As shown in Fig. 3b , after reaction of 6 h, the 13 C NMR spectrum clearly displays three peaks at 125.7, 159.8, and 164.4 ppm, corresponding to CO 2, HCO 3 − , and HCOO − respectively. In contrast, these three peaks were absent in the 13 C NMR spectrum when 12 CO 2 was used as the reactant (Supplementary Fig. 17 ), unambiguously demonstrating that Eu-Ru(phen) 3 -MOF indeed promotes the photocatalytic CO 2 reduction. In the photocatalytic reaction, TEOA were oxidized to its aldehyde form (Supplementary Figs. 18 and 19 , Supplementary Note 2 ). Absorption and PL analyses To reveal the photoinduced charge transport mechanism, we investigated the samples by using Ultraviolet–visible (UV–vis) absorption, static, and time-resolved emission spectra. As shown in Fig. 4a , Eu-Ru(phen) 3 -MOF and H 3 L both showed strong absorption bands at 300–350 nm because of the π–π* transition of phen ligand. The relatively weaker absorption peaks in the region of 420–480 nm correspond to the characteristic broad absorption of Ru 2+ -centered metal-to-ligand charge transfer (MLCT) transitions. This similarity between H 3 L ligand and MOF suggested that the coordination of Eu 3+ with H 3 L has no significant effect on the excitation energy of the latter [34] , [35] . However, the emission of H 3 L centered at ~590 nm, which represents the Ru(phen) 3 -centered triplet 3 MLCT state, is significantly quenched after Eu 2 coordination in MOF (Fig. 4a ). Consistently, the time-resolved PL collected in the time window of <1 ns to 15 μs (Fig. 4b ) of MOF shows much faster decay kinetics than H 3 L . These results suggest possible electron and/or energy transfer from H 3 L to Eu 2 oxo-clusters [36] . Notably, no characteristic Eu 3+ f – f emission were observed in Eu-Ru(phen) 3 -MOF, implying that the quenching and fast decay of Eu-Ru(phen) 3 -MOF emission should be due to electron transfer rather than energy transfer from H 3 L to Eu f – f transitions. To quantitatively estimate the electron transfer rate, the time-resolved PL kinetics are fitted by a bi-exponential function, as shown in Supplementary Tables 2 and 3 . An electron transfer time ranging from 6.1 ns to 293.6 ns is determined (Supplementary Note 3 ). Fig. 4 Spectroscopic evidence for effective electron transfer process. a Normalized UV–vis of Eu-Ru(phen) 3 -MOF and H 3 L in DMF. Inset: Emission spectra of Eu-Ru(phen) 3 -MOF and H 3 L ( λ ex = 465 nm). b Normalized luminescence decay traces of Eu-Ru(phen) 3 -MOF and H 3 L over the first 50 ns ( λ ex = 377 nm). Inset: Decay transients measured at 630 nm ( λ ex = 465 nm). c Transient absorption spectra of Eu-Ru(phen) 3 -MOF and H 3 L at various time delays, and d corresponding kinetic traces at 604 nm Full size image Ultrafast transient absorption and EPR characterizations To further confirm the photoinduced electron transfer kinetics in MOF, ultrafast transient absorption (TA) measurements were also carried out (the details of TA experiments in Supplementary Methods) [37] , [38] , [39] . In Fig. 4c , we show the comparison of the TA spectra between H 3 L ligand and Eu-Ru(phen) 3 -MOF at different delay times after 400 nm excitation. The TA spectra of H 3 L exhibits negative ground state bleach (GSB) signal at ~440 and ~490 nm, which overlaps with a strong and broad (440–700 nm) excited state absorption (ESA) signal (positive). In contrast, the ESA amplitude is significantly reduced in the MOF sample, leaving a more prominent and long-lived GSB signal. This spectroscopic feature further confirms the electron transfer from H 3 L to the coordinated Eu metal node rather than energy transfer, because in the latter case the GSB recovery and ESA decay should occur simultaneously. The TA kinetics of H 3 L and MOF probed at ESA (604 nm) are shown in Fig. 4d . The ESA signal in MOF shows a considerably faster decay, which reflects the electron transfer process. 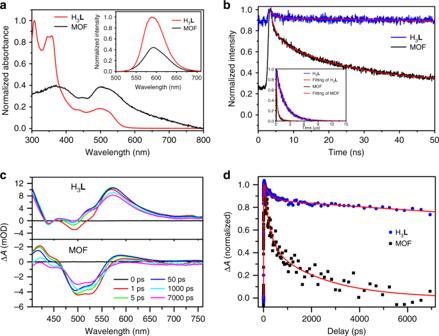Fig. 4 Spectroscopic evidence for effective electron transfer process.aNormalized UV–vis of Eu-Ru(phen)3-MOF and H3Lin DMF. Inset: Emission spectra of Eu-Ru(phen)3-MOF and H3L(λex= 465 nm).bNormalized luminescence decay traces of Eu-Ru(phen)3-MOF and H3Lover the first 50 ns (λex= 377 nm). Inset: Decay transients measured at 630 nm (λex= 465 nm).cTransient absorption spectra of Eu-Ru(phen)3-MOF and H3Lat various time delays, anddcorresponding kinetic traces at 604 nm By fitting the kinetics by a bi-exponential function (Supplementary Table 4 ), we determined the electron transfer time of 1.2 ns. This transfer time is consistent with the faster time rate observed in time-resolved PL measured within 50 ns windows (Fig. 4b ). The results of TA and time-resolved PL indicate that the electron transfer from H 3 L to the Eu 2 oxo-clusters occurs on a broad time scale, ranging from a nanosecond to hundreds of nanosecond (Fig. 5a ). However, according to the significant change of ESA signal in TA spectra, which decays by 90% in MOF vs. 20% in H 3 L , the electron transfer process should occur mainly within a few nanosecond time, which is consistent with reported electron transfer time in similar Ru–Pt complex [40] . Nevertheless, the observation of a wide range of electron transfer time suggest that the electron transfer process in Ru(phen) 3 -MOF may occurs along different transport pathways. Fig. 5 Photocatalytic in situ EPR characterization. a Schematic light-induced dynamics of Eu-Ru(phen) 3 -MOF based on the initial excitation of the Ru photocenter and the pathways of electron transfer from Ru to catalytic Eu 2 oxo-cluster center. b In situ EPR spectra of Eu-Ru(phen) 3 -MOF under different conditions Full size image Following the electron transfer process for H 3 L ligand to the Eu metal, the recovery of GSB in the TA spectra of MOF sample reflects the back electron transfer from Eu metal node to H 3 L ligand, which brings the H 3 L cation to ground state. Within our TA time window of 7 ns, GSB signal recovers by only 30%, suggesting that the back electron transfer time is much longer than 7 ns. The slow back electron transfer thus ensures an effective charge separation in the MOF for CO 2 reduction. To obtain further insight into the photocatalytic process of CO 2 reduction, in situ EPR experiments were studied as well, which can elucidate the photo-induced electron injection process. Under visible-light irradiation in a N 2 atmosphere, the EPR spectrum of H 3 L shows a signal at g = 2.04. Meanwhile, when the light source was turned off, the signal quenching was observed immediately reflecting the visible-light-induced radical formation of the metalloligand and the subsequent charge transfer process (Supplementary Fig. 20 ). For Eu-Ru(phen) 3 -MOF, no EPR signal was observed without irradiation. Upon 2 min of visible-light irradiation, a broad EPR signal with g = 2.23 was observed, simultaneously a weak EPR signal was found at 4.61 (Fig. 5b ). These two EPR signals are attributed to paramagnetic Eu 2+ species, because the Eu 3+ ions have no EPR signals, while the Eu 2+ ions are EPR active [41] , [42] . The valence change of the Eu 2 oxo-clusters can be attributed to the photo-induced LMCT process. Subsequently, when CO 2 was introduced into the irradiated Eu-Ru(phen) 3 -MOF, the EPR signal corresponding to Eu 2+ was greatly weakened due to some of the Eu 2+ oxidized back to Eu 3+ during the CO 2 reduction process. DFT calculations To probe the active site of Eu-Ru(phen) 3 -MOF, the spin polarized density functional theory (DFT) calculations were studied using VASP program with Hubbard U correction ( Supplementary Methods ) [43] , [44] . In order to optimize the structure of Eu-Ru(phen) 3 -MOF, all hydrogen atoms were relaxed under the constraint of non-hydrogen atoms. The Eu 2 unit derived from the structure was used as the computational model. The optimized structure reflects the Eu1-Ow1 bond that is weaker than the others, with an enthalpy difference of 0.80 eV. Therefore, removal of the Ow1 can generate a Lewis acid site of Eu(III), which is possibly facilitated by visible-light irradiation. The exposed Eu(III) center can adsorb one CO 2 molecule through Eu-O linkage. Figure 6a illustrates the position of the CO 2 adsorbed on the active site of Eu1 ion ( d (Eu1-O) = 2.745 Å), which was obtained from geometry optimization using DFT. 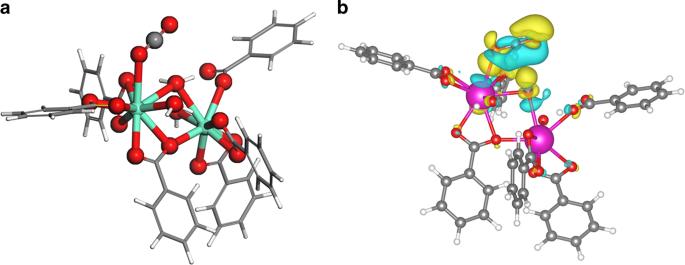Fig. 6 Density functional theory calculation.aThe calculated CO2adsorption structure.bCharge difference density of CO2adsorption structure of Eu(II)2 The adsorption energy of CO 2 was estimated to be −0.55 eV. After reducing the Eu(III) to Eu(II) via photo-induced electron injection, electron can be further transferred to CO 2 . The difference map of charge density reveals that CO 2 molecule can obtain 0.025 electrons from the Eu(II) 2 dimer (Fig. 6b ) [45] , while Eu(II)1 and Eu(II)2 ions lose 0.0073 and 0.004 electrons, respectively, suggesting an effective activation of CO 2 molecule. Fig. 6 Density functional theory calculation. a The calculated CO 2 adsorption structure. b Charge difference density of CO 2 adsorption structure of Eu(II) 2 Full size image To investigate the photocatalytic mechanism, photophysical and electrochemical studies were performed. To establish whether the excited [Ru II (phen) 3 ] 2+ was quenched reductive by TEOA or oxidative by Eu 2 clusters, the luminescence quench experiments of H 3 L was studied with addition of the solution of TEOA or Eu 2 clusters in DMF. The discrete Eu 2 clusters with a similar structure to that of Eu 2 SBUs in Eu-Ru(phen) 3 -MOF can be synthesized with a formula of [Eu 2 (MMA) 6 (H 2 O) 4 ] (MAA = methacrylic acid) [46] (Supplementary Fig. 21 and Supplementary Methods). As shown in Fig. 7a , the luminescence of H 3 L was quenched by the Eu 2 moieties efficiently but not by TEOA (Fig. 7b ). These results indicated that the photocatalytic reduction of CO 2 process occurred via electron transfer from the photoexcited [Ru II (phen) 3 ] 2+ to Eu 2 SBUs, but not from TEOA to the excited [Ru II (phen) 3 ] 2+ . In the oxidative quenching, the generated [Ru III (phen) 3 ] 3+ was reduced by TEOA subsequently. Fig. 7 Fluorescence quenching. a Emission spectra of H 3 L after the addition of different amounts of [Eu 2 (MMA) 6 (H 2 O) 4 ] and b TEOA in DMF with 465 nm excitation Full size image On the other hand, to investigate the thermodynamic parameters and the driving force for the reduction of CO 2 , we measured the reduction potentials of the Eu 2 SBUs and calculated the energy of {[Ru II (phen) 3 ]}* excited state, which can provide additional insight into the photocatalytic reaction. The cyclic voltammograms (CVs) of dinuclear Eu 2 compound shows a reversible peak at −0.69 vs. NHE (Supplementary Fig. 22 ). The reduction potential of Eu III /Eu II is more negative than that of CO 2 /HCOOH (−0.58 V vs. NHE). Furthermore, the energy difference Δ E 1 between excited state of {[Ru II (phen) 3 ]}* and ground state of {[Ru II (phen) 3 ]} can be calculated from the luminescence emission peak at 598 nm (Δ E 1 = 2.07 eV, Supplementary Fig. 23a ). In addition, as shown in Supplementary Fig. 23b , the CVs of H 3 L showed the redox potential of [Ru III (phen) 3 ] 3+ /[Ru II (phen) 3 ] 2+ to be 1.19 V vs. NHE (−Δ E 3 ). Based on the energy loop (Fig. 8 ), the redox potential Δ E 2 of {[Ru II (phen) 3 ]}*/[Ru III (phen) 3 ] 3+ was calculated to be −0.88 V vs. NHE (Δ E 2 = 1.19–2.07 eV), which is more negative than the −0.69 V of the Eu 2 SBUs to drive the reduction of Eu 2 SBUs. These results indicate that under photocatalytic conditions, the {[Ru II (phen) 3 ]}* transfer electrons to [Eu III -H 2 O-Eu III ] unit, resulting in the reduced [Eu II -H 2 O-Eu II ] unit, which then transfers electrons to CO 2 for its reduction. Fig. 8 Proposed catalytic mechanism of photocatalytic CO 2 reduction to HCOOH. The photo-initiated electron transfers from Ru photocenters to dinuclear Eu 2 oxo-clusters in Eu-Ru(phen) 3 -MOF lead to the photo-reduction of CO 2 . Δ E 1 = 2.07 eV, Δ E 2 = −0.88 eV, Δ E 3 = −1.19 eV, and Δ E’ = −0.69 eV Full size image In light of the above experimental results and DFT calculations, the photocatalytic mechanism is proposed (Fig. 8 ). Under the visible-light irradiation, the ligand [Ru II (phen) 3 ] will be excited to triplet MLCT excited state, {[Ru II (phen) 3 ]}*, which can transfer one electron to the [Eu III -H 2 O-Eu III ] unit through multistep relaxation and afford [Ru III (phen) 3 ]. Consequently, the [Eu III -H 2 O-Eu III ] unit accepted two electrons from two adjacent [Ru II (phen) 3 ] to give dinuclear [Eu II -H 2 O-Eu II ] active site, which can selectively reduce CO 2 to HCOOH in a two-electron process. Finally, the [Ru III (phen) 3 ] can be reduced back to the [Ru II (phen) 3 ] by sacrificial donor (TEOA) to complete the catalytic cycle. Additionally, as shown in Supplementary Figs. 24 – 26 , energy levels of the metalloligand and Eu 2 node that are involved in the electron–hole separation process were determined with a combination of optical absorption spectra analysis and electrochemical measurements (Supplementary Note 4 ). In summary, we demonstrate a photosensitizing MOF based on {Eu(III)} 2 cluster and Ru(phen) 3 -derived ligand, featuring high photocatalytic activity for visible-light-driven CO 2 reduction. Remarkably, the efficient electron transfer from Ru(phen) 3 -derived tricarboxylate ligand to {Eu(III)} 2 catalytic centers allowed high formate production rate of 321.9 μmol h −1 mmol MOF −1 . The in situ photo-generated dinuclear [Eu II -H 2 O-Eu II ]-active sites are involved in two-electron reduction of CO 2 to selectively produce HCOOH. This work not only provides a strategy to design and synthesize highly effective photocatalytic catalysts based on lanthanide cluster but also provides a platform for understanding the electron transfer mechanism in Ln-MOF materials. Materials and equipment Unless otherwise mentioned, all starting materials and chemicals were purchased from commercial vendors and used without further purification. Crystallographic data of Eu-Ru(phen) 3 -MOF was collected on a MarCCD mx300. The PRXD data were collected on Agilent SuperNova (Rigaku) with CuKα radiation sources (15 mA, 40 kV). 1 H-NMR 1 H- 1 H COSY and 13 C NMR spectra were recorded on a Bruker NMR 500 DRX spectrometer at 500 MHz. The 13 C spectra were referenced to DMSO- d 6 (δ = 39.52). Mass spectrum was recorded on an Agilent Technologies ESI-MS in CH 3 CN. ICP-MS data were obtained with an Agilent 7700x ICP-MS and analyzed using ICP-MS MassHunter version B01.03. Samples were decomposed by 68% HNO 3 and then diluted to a 2% HNO 3 solution and analyzed with a 159 Tb internal standard against a 10-point standard curve. The correlation coefficient was >0.9997 for all analytes of interest. TGA experiment was performed on an SDT Q600 thermal analysis system and the samples were heated from 30 to 800 °C with a slow rate of 10 °C min −1 under N 2 . SEM studies were performed on ZEISS SIGMA. Fluorescence spectra were taken at room temperature on Hitachi F7000 and the time-resolved PL experiments were carried out on an Edinburgh FLS980 fluorescence spectrometer. Gas sorption measurement was performed on a Micromeritics ASAP 2020 system at desired temperatures. UV–Vis studies were carried out on a UV-2401 PC UV–Vis recording spectrometer. EPR spectra were recorded on Bruker EMX-10/12 EPR spectrometer. Synthesis of Eu-Ru(phen) 3 -MOF Eu(NO 3 ) 3 ·6H 2 O (42.0 mg, 94.2 µmol), H 3 L (8.0 mg, 7.1 µmol), 2-FBA (100 mg, 0.719 mmol), and DMF (3 mL) was sealed in a 20 mL Telfon-lined autoclave, and then heated to 105 °C for 70 h in a preheated oven. After cooling down to room temperature, the red block-shaped crystals (3 mg, 44% yield) were obtained. Formula of MOF: [Eu 2 (μ 2 -H 2 O)(H 2 O) 3 (L) 2 ]·(NO 3 ) 2 ·(2-FBA) x ·(H 2 O) y ( x ≈ 2, Y ≈ 22). The NO 3 − counter anions, guest water molecules, and 2-FBA are severely disordered and therefore removed by SQUEEZE method using the PLATON software. The number of the NO 3 − counter anions, guest water molecules, and 2-FBA were confirmed by charge balance, element analysis, and thermogravimetric analysis. Anal. Calcd. For Eu 2 Ru 2 H 126 C 134 N 26 F 2 O 48 (FW = 3412.65, based on two 2-FBA and 22 H 2 O guest molecules): C, 47.16, H, 3.72, N, 10.67, Found: C, 47.07, H, 3.74, N, 10.35. Single-crystal X-ray diffraction determination of Eu-Ru(phen) 3 -MOF Data of the Eu-Ru(phen) 3 -MOF was collected on a MarCCD mx300 at 100 K in the National Center for Protein Sciences Shanghai at the Shanghai Synchrotron Radiation Facility. Block-shaped single crystal of Eu-Ru(phen) 3 -MOF was chosen under a microscope on a plastic fiber loop for measurement. Data reduction and integration were performed with the HKL3000 software. The wavelength of X-ray corrections were performed using program of PLATON. The structures were solved by direct methods and refined to convergence by least-squares method on F 2 using the SHELXTL software. The disordered guest water molecules and 2-FBA in structure of MOF were removed by using the PLATON software with SQUEEZE method. 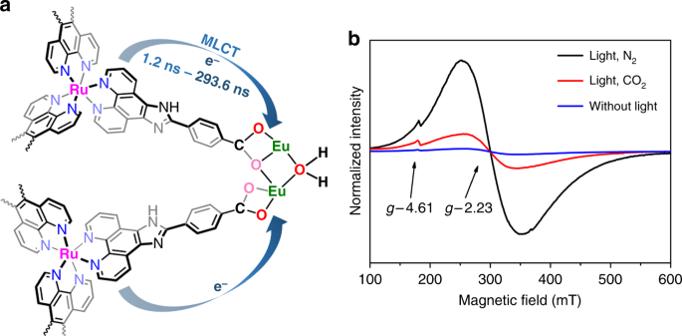In addition, hydrogen atoms are refined isotropically. Fig. 5 Photocatalytic in situ EPR characterization.aSchematic light-induced dynamics of Eu-Ru(phen)3-MOF based on the initial excitation of the Ru photocenter and the pathways of electron transfer from Ru to catalytic Eu2oxo-cluster center.bIn situ EPR spectra of Eu-Ru(phen)3-MOF under different conditions Cambridge Crystallographic Data Center (CCDC) number of 1576282 for MOF contains the supplementary crystallographic data that is summarized in Supplementary Table 5 . Femtosecond TA spectroscopy The TA measurements were carried out on a regenerative amplified Ti:sapphire laser system in combination with nonlinear frequency mixing techniques and the ultrafast TA spectrometer (Time-Tech Spectra, femtoTA100) [47] . During the measurements, samples under investigation were dispersed in DMF and placed in a 2 mm quartz curvette with stirring by a magnetic stirrer, constantly. Detailed procedures for the femtosecond TA measurements can be found in the Supplementary Methods . Photocatalytic reactions The photocatalytic activities of the samples were performed via a controllable reaction system (CEL-SPH2N, CEAULight, China) with a volume of approximately 300 mL. The setup of the photocatalytic system is shown in Supplementary Fig. 12 . The mixture of catalyst MOF 50 mg or H 3 L 50 mg, TEOA (2.0 mL), and CH 3 CN (40.0 mL) was sealed in a 100 mL Pyrex flask. To remove the dissolved oxygen, the flask was capped with a quartz septum and degassed with a pure CO 2 for 30 min. The light source is a 300 W xenon lamp through a UV cut filter with a wavelength range of 420–800 nm. The HCOO − in liquid phase was quantified by an ion chromatography (881 Compact IC pro, Metrosep) with a Metrosep A supp 5 250/4.0 column under 303 K. In addition, the eluent is the mixed solution of NaHCO 3 (1000 μM) and Na 2 CO 3 (3200 μM). Gas productions were performed on a gas chromatograph (Aulight GC-7920) equipped with a thermal conductivity detector (TCD) and flame ionization detector (FID). After each reaction time, the evolved gaseous phase in the headspace of the Pyrex flask was sampled with a gastight syringe (500 µL) and measured by GC (N 2 as a carrier gas) using the TCD (a packed column with molecular sieves 5 A (3.0 m × 3.0 mm, 60–80 mesh) at 373 K) to detect H 2 and using the FID (a column (TDX-1, 3.0 m × 0.30 mm) at 653 K) to detect CH 4 and CO. However, no signals for H 2 , CH 4 , and CO can be observed. 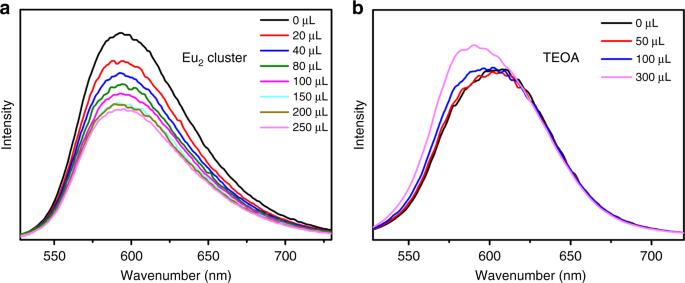Fig. 7 Fluorescence quenching.aEmission spectra of H3Lafter the addition of different amounts of [Eu2(MMA)6(H2O)4] andbTEOA in DMF with 465 nm excitation 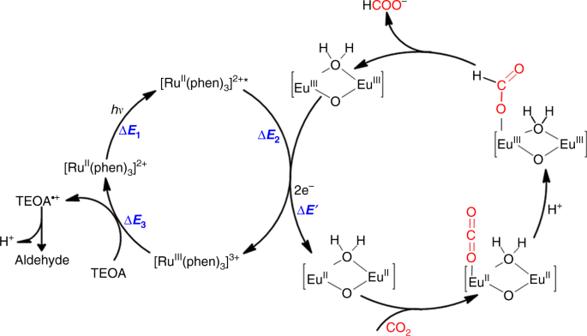Fig. 8 Proposed catalytic mechanism of photocatalytic CO2reduction to HCOOH. The photo-initiated electron transfers from Ru photocenters to dinuclear Eu2oxo-clusters in Eu-Ru(phen)3-MOF lead to the photo-reduction of CO2. ΔE1= 2.07 eV, ΔE2= −0.88 eV, ΔE3= −1.19 eV, and ΔE’= −0.69 eV In situ EPR experiments The in situ EPR experimental data were obtained over a commercial EPR spectrometer Bruker EMX-10/12 at a X-band (9 GHz). Samples were prepared by mixing the catalyst in a glass tube with 0.5 mL solution of CH 3 CN/TEOA (20:1). The sample was degassed by N 2 and then sealed. Then the glass tube was fixed into the EPR resonator. When needed, the CO 2 were introduced into the sample. The experiments were performed under visible-light irradiation. Data availability The X-ray crystallographic data for structure Eu-Ru(phen) 3 -MOF has been deposited at the CCDC, with a CCDC number of 1576282. The data can be obtained free of charge from The Cambridge Crystallographic Data Centre via www.ccdc.cam.ac.uk/data_request/cif . All other data supporting the findings of this study are available within the article and its Supplementary Information files , or from the corresponding author on reasonable request.